Roaming dynamics in radical addition–elimination reactions Radical addition–elimination reactions are a major pathway for transformation of unsaturated hydrocarbons. In the gas phase, these reactions involve formation of a transient strongly bound intermediate. However, the detailed mechanism and dynamics for these reactions remain unclear. Here we show, for reaction of chlorine atoms with butenes, that the Cl addition–HCl elimination pathway occurs from an abstraction-like Cl-H-C geometry rather than a conventional three-centre or four-centre transition state. Furthermore, access to this geometry is attained by roaming excursions of the Cl atom from the initially formed adduct. In effect, the alkene π cloud serves to capture the Cl atom and hold it, allowing many subsequent opportunities for the energized intermediate to find a suitable approach to the abstraction geometry. These bimolecular roaming reactions are closely related to the roaming radical dynamics recently discovered to play an important role in unimolecular reactions. Chlorine atom reactions with alkenes are an important prototype for the broad class of radical addition–elimination reactions: chlorine sources literally cover the Earth with both oceanic and anthropogenic origins and alkenes are among the most abundant atmospheric hydrocarbons [1] . These reactions play an important role in the oxidation of volatile organic compounds in marine boundary layers and the Polar regions [2] , [3] , [4] , the burning of hazardous waste [5] and possibly the aging of organic aerosols by heterogeneous processes [6] . In these bimolecular reactions that have become key in studying polyatomic reaction dynamics both in the gas phase [7] and in solution [8] , HCl formation is a major pathway for which addition–elimination competes with direct abstraction: Direct abstraction and addition–elimination exhibit identical exoergicity (15–30 kcal mol −1 ) and their decomposition is a long-standing challenge in both kinetics and dynamics studies for the obvious reason that they give rise to the same products. Nowadays, the kinetics of numerous Cl+alkene reactions seem to be well understood, with the gas-phase reactions exhibiting rate constants close to the gas kinetic limit, while evidence has been shown for addition–elimination involving a long-lived C n H 2 n Cl intermediate [9] , [10] , [11] , [12] . However, the details of the reaction mechanism and dynamics remain unknown. State-selected HCl measurements have not shown a distinct feature of addition–elimination in the product distributions [13] . Quantum chemical calculations of reaction potential energy surfaces (PESs) have been unable to corroborate the addition–elimination mechanism [14] , [15] . Recently, we have investigated the reactions of chlorine atoms with various alkenes such as butene isomers, 1-pentene and various hexene isomers using a crossed-beam apparatus coupled to DC slice ion imaging [16] , [17] We have found that the scattering distributions reflect the competition between direct H abstraction and Cl addition–HCl elimination. Our earlier preliminary theoretical calculations did not locate any typical transition states (TSs) for HCl elimination, for example, three-centre or four-centre TSs such as are generally seen for HCl elimination from closed-shell halides. This suggested the possibility that the decomposition of the C 4 H 8 Cl complexes might occur via a roaming radical mechanism [18] . Roaming dynamics are now widely recognized as an important pathway in unimolecular reactions [19] , [20] , [21] , [22] but their role in bimolecular reactions remains an open question. In this work we show specifically for the case of Cl with isobutene that addition–elimination occurs by a mechanism involving Cl atom roaming. Imaging Cl+isobutene dynamics in crossed beams Our experimental approach consists in probing the hydrocarbon radical product in crossed molecular beams, and is therefore complementary to state-resolved HCl detection. For this study, pulsed supersonic beams containing atomic chlorine and isobutene seeded in rare gases were crossed at 90° under single-collision conditions. The interaction region was illuminated by an F 2 excimer laser beam at 157 nm (hν=7.9 eV), directly ionizing the C 4 H 7 alkenyl product. The recoiling ions were then accelerated onto a position-sensitive detector, viewed by a charged-coupled device camera, which was gated to detect the C 4 H 7 + mass products scattered in the plane of the molecular beams and parallel to the detector. After image accumulation, background subtraction and density-to-flux correction, the images yield the velocity-flux contour maps, which embody coupled translational energy P(E T ) and angular T(Θ) centre-of-mass distributions for the reaction. The choice of isobutene as a target system should be noted before going into details of the reactive scattering distributions. There are two different sites that can lead to the formation of HCl and the alkenyl radical: The first one, the vinylic site, is directly located on the less substituted sp 2 carbon atom; the second one, the allylic site, is located on the two methyl groups adjacent to the double bond. Reactions at the allylic sites are thermodynamically very favourable with enthalpies of reaction ΔrH(0 K)~\n−16 kcal mol −1 , while H removal by Cl at the vinylic site is an endoergic process with ΔrH(0 K)~\n7 kcal mol −1 (ref. 17 ). The latter reaction is therefore unlikely to occur under our experimental conditions, although the highest collision energy could permit this reaction. Moreover, we use an unfocused probe laser in our present experimental configuration that avoids any non-resonant multiple photon ionization of the products. Given the ionization energies of the two possible product radicals (ionization energies of allylic and vinylic C 4 H 7 radicals are ~\n7.9 (ref. 23 ) and 8.4 eV, respectively, with the latter value calculated at the CBS-QB3 level of theory), and the fact that H migration cannot occur in the energized radical product as established for similar systems (propene and isoprene) [15] , we can confidently rule out the possible detection of radical products stemming from the abstraction directly at the double bond. The distributions presented here, and their changes with collision energies, correspond to reaction at the allylic sites only. Direct versus addition–elimination pathways Direct and indirect pathways for HCl production will appear very differently in the scattering distributions as illustrated in Fig. 1 . The product direction is taken as zero for the case of no momentum transfer, which corresponds in our case to the hydrocarbon beam direction. On this basis, we define for the radical product three different angular components in the centre-of-mass frame, namely forward (FW, 0–60°), sideways (SW, 60–120°) and backward (BW, 120–180°). For direct H abstraction, the mechanistic picture is similar to the one in Cl+alkane reactions [24] , [25] . The rebound component, associated to modest rotational and vibrational excitation, gives reactive scattering in the BW–SW directions; the stripping component involves little energy and momentum transfer, and appears in the FW scattering direction. In all cases the direct reaction will tend to show translational energy release similar to the initial collision energy owing to the kinematics of H atom transfer. Moreover, for the direct reactions, the forward scattered distribution is sharply peaked and its intensity typically grows with collision energy as the fraction of the stripping component grows. Formation of a long-lived adduct shows very distinct scattering distributions: randomization of the internal energy over the vibrational degrees of freedom in the complex leads to product translational energy distributions that peak at low energy. Moreover, if the complex lifetime is significantly longer than its rotational period, the system loses reference to the initial approach direction: the angular distributions show scattering that is symmetric in the FW and BW directions and the translational energy distributions in all directions will be identical. For systems in which the scattering is non-planar (such as often the case in more complex polyatomic systems), this symmetric scattering becomes fully isotropic. 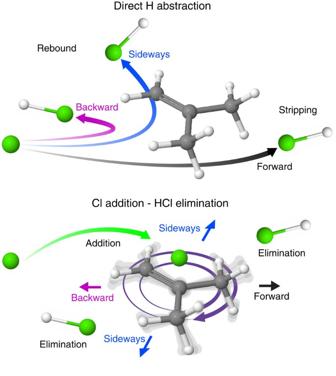Figure 1: Cartoon illustrating the reaction dynamics Cl+alkene reactions. Direct H abstraction and addition–elimination are contrasted for Cl reaction with the isobutene molecule. The reactive scattering components measured in the crossed-beam imaging set-up, namely forward, sideways and backward, are highlighted. Figure 1: Cartoon illustrating the reaction dynamics Cl+alkene reactions. Direct H abstraction and addition–elimination are contrasted for Cl reaction with the isobutene molecule. The reactive scattering components measured in the crossed-beam imaging set-up, namely forward, sideways and backward, are highlighted. Full size image The centre-of-mass angular and translational energy distributions for reaction of Cl ( 2 P 3/2 ) with isobutene for collision energies of 14, 8 and 4 kcal mol −1 are shown in Fig. 2 . In this case we see evidence of both characteristic distributions. At E C =14 kcal mol −1 , the translational energy distribution in the FW direction peaks at substantially higher energy than in the SW and BW distributions, and the angular distribution shows a minimum around 90° and a modest enhancement of the FW scattering. This immediately indicates some direct component in the reaction, showing features reminiscent of the distributions observed for Cl+alkane reactions in this collision energy range. At the intermediate collision energy, the angular distribution is slightly flattened, showing an evolution towards a more isotropic reactive scattering with decreasing collision energy. The distinction between the FW and SW/BW distributions is less pronounced and the BW translational energy release peaks at ~\n20% of the collision energy. At E C =4 kcal mol −1 , the translational energy release peaks near 0 kcal mol −1 and the angular distribution is fully isotropic, although the centre-of-mass is brought closer to the photochemical background and reliable data in the FW direction cannot be obtained. Nevertheless, these distributions tell a clear story. The complex-mediated mechanism plays a prominent role in these reactions, although it is not possible to decompose the precise relative contributions of direct versus indirect reactions from these experiments. 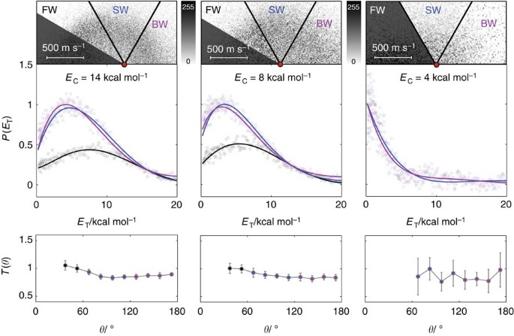Figure 2: Centre-of-mass distributions of the C4H7radical for different collision energies. Translational energy distributions P(ET) and angular distributions T(Θ) are plotted for forward (30–60°, black), sideways (60–120°, blue) and backward (120–180°, purple) scattered products. The P(ET) are fitted by least squares polynomial regressions. The T(Θ) are shown averaged every 15° with error bars estimated by mean absolute deviation of the raw data in the corresponding angle range. The corresponding velocity-flux contour maps are shown with the photochemical background masked. The red spots correspond to the centres-of-mass at the three different collision energies. Figure 2: Centre-of-mass distributions of the C 4 H 7 radical for different collision energies. Translational energy distributions P(E T ) and angular distributions T(Θ) are plotted for forward (30–60°, black), sideways (60–120°, blue) and backward (120–180°, purple) scattered products. The P(E T ) are fitted by least squares polynomial regressions. The T(Θ) are shown averaged every 15° with error bars estimated by mean absolute deviation of the raw data in the corresponding angle range. The corresponding velocity-flux contour maps are shown with the photochemical background masked. The red spots correspond to the centres-of-mass at the three different collision energies. Full size image The question now is the pathway for the decomposition of the adduct. Here the translational energy distributions can provide insight. If the HCl elimination involved a conventional three-centre or four-centre TS, we would expect to see the translational energy distribution peak away from zero as the strained TS geometry relaxes to products. Instead we find, at the lowest collision energy, only 10% of the available energy appears in translation. This implies no experimental evidence for a conventional TS mediating the elimination, and this is strongly supported by the theoretical calculations below. We can also ask where the missing energy might be found. Pilgrim and Taatjes [12] measured the HCl vibrational energy disposal in the Cl+propene reaction and found that significant amount of reaction exothermicity (28±3%) was channeled into HCl vibration with half of the population in vibrationally excited levels [12] . We expect a similar result here, and little total energy in rotation, implying that the greatest fraction of the unaccounted energy is retained in the internal energy of the hydrocarbon radical itself, holding >60% of the energy available for addition–elimination reactions. Again, this is the anticipated result for decomposition of a complex given the large number of internal degrees of freedom of the radical product. Properties of the addition complex We now turn the discussion on the PES. Ab initio calculations were performed using the CBS-QB3 method [26] , which provides a thermochemical accuracy of ~\n2 kcal mol −1 . The key stationary points (minima and TSs) for the Cl+isobutene reaction are shown in Fig. 3 . Direct H abstraction is exoergic by 16.2 kcal mol −1 at the allylic sites and endoergic by 7.3 kcal mol −1 at the vinylic site. Our calculations show that when Cl approaches isobutene from the side of the methyl groups, HCl elimination proceeds without any barrier. We also find there exist van der Waals C 4 H 7 …HCl complexes, which are bound by 2.6 kcal mol −1 . The absence of barriers was confirmed via a careful scan of the minimal energy reaction path through partial geometry optimization with the critical H–Cl and C–H distances being frozen for the entrance channel and the exit channel, respectively. For reaction at the vinylic site, no TS has been located. 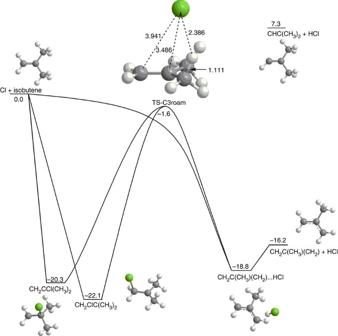Figure 3: Key points on the PES of the Cl+isobutene reaction. Direct H abstraction is a barrierless pathway with a van der Waals complex in the exit channel. The two addition complexes undergo near dissociation to reach a unique roaming-type TS (TS-C3roam) before eliminating HCl. The diagram has been calculated at the CBS-QB3 level of theory. Relative energies are shown in kcal mol−1. Figure 3: Key points on the PES of the Cl+isobutene reaction. Direct H abstraction is a barrierless pathway with a van der Waals complex in the exit channel. The two addition complexes undergo near dissociation to reach a unique roaming-type TS (TS-C3roam) before eliminating HCl. The diagram has been calculated at the CBS-QB3 level of theory. Relative energies are shown in kcal mol −1 . Full size image The roaming TS The reaction can also proceed by barrierless addition of the Cl atom to C1 or C2 carbons leading to H 2 CClC(CH 3 ) 2 or H 2 CCCl(CH 3 ) 2 radicals, residing in deep potential wells of 20–22 kcal mol −1 . Similar to the previous theoretical studies of Cl reactions with propene [11] and isoprene [12] , we could not locate ‘conventional’, tight TSs for HCl elimination from the chlorobutenyl complexes. The reason for this is likely to be the same as for the absence of tight TSs for H 2 addition to radicals [27] , [28] and may be understood on the basis of simple orbital symmetry arguments. For example, when H 2 adds to vinyl radical, electron density must be donated from the singly occupied p orbital to the antibonding σ u orbital in H 2 , the most favourable interaction being in the collinear abstraction geometry. It was proposed that this may be a general feature of H 2 addition to radicals with an unpaired p -electron, and similar arguments would apply to the reverse reactions of H 2 elimination or HCl elimination considered here. Although no tight TSs were found, we were able to find pathways connecting these strongly bound C 4 H 8 Cl intermediates with the allylic C 4 H 7 +HCl product channel. The structure of the TS along the addition–elimination pathway, shown in Fig. 3 , is peculiar. The Cl–H distance for the forming H–Cl bond is 2.366 Å with the corresponding attacked C–H bond stretched only to 1.111 Å. The Cl atom is 3.468 and 3.941 Å away from C2 and C1 carbons, respectively. According to intrinsic reaction coordinate (IRC) calculations ( cf . Fig. 4 ), the TS is connected to the van der Waals H 2 CCCH 3 CH 2 …HCl product complex. In the reverse direction, IRC calculations return back to the C2 addition complex. However, as the Cl atom is located far from both C1 and C2, the downhill pathway from the TS may also bifurcate to the C1 addition complex. Therefore, the Cl addition–HCl elimination TS is both early, because the H–Cl bond barely starts to form and the breaking C–H bond is only slightly stretched, and late, because the C–Cl bond is already broken. Based on its structure and the IRC path, this TS is typical for a roaming radical mechanism, in which the Cl atom unlinks from the CC double bond, is about to be eliminated (returning to reactants), but wanders in the direction of the allylic site and picks up a hydrogen from a methyl group to form HCl. This observation is corroborated by vibrational frequencies computed for the TS, which include a low imaginary frequency (317 cm −1 ), two very low bound frequencies corresponding to motions of the Cl atom relative to the isobutene fragment (45 and 78 cm −1 ) with the remaining frequencies being very similar to those of isobutene. The only exception is one C–H stretching frequency, which is reduced to 2,706 cm −1 because this bond is slightly elongated and thus begins to break in the TS as the H atom is being abstracted by the roaming Cl radical. We have performed similar calculations for Cl reaction with all other butene isomers. Only roaming-type TSs for addition–elimination were found, although the PESs were complicated by additional H abstraction sites. 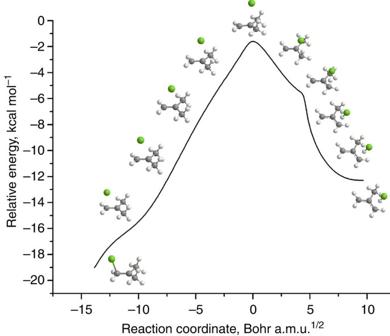Figure 4: Lowest energy pathway linking the C1 addition complex and HCl elimination. Potential energy is plotted as a function of the IRC with respect to the dissociation asymptote. Calculations are carried out at the B3LYP/6-311 G(2d,d,p) level of theory. Relative energies are shown in kcal mol−1. Figure 4: Lowest energy pathway linking the C1 addition complex and HCl elimination. Potential energy is plotted as a function of the IRC with respect to the dissociation asymptote. Calculations are carried out at the B3LYP/6-311 G(2d,d,p) level of theory. Relative energies are shown in kcal mol −1 . Full size image Based on the TS structure shown in Fig. 3 , both addition–elimination and abstraction mechanisms should be expected to produce HCl with similar vibrational excitation. The HCl product vibrational distributions may therefore not be helpful for distinguishing between the direct and indirect reaction pathways. The statistical lifetimes of the Cl complexes on dissociation, estimated from energy-dependent rate constant calculations based on the Rice–Ramsperger–Kassel–Marcus theory [29] , are too long at both low and high energies (72 and 2 ns, respectively) to account for the onset of the FW component when compared with the rotational period (~\n30 ps) of the complex. This observation, combined with the observed shift in the translational energy distribution in the FW direction suggests that it is the appearance of the direct reaction at higher collision energy, bypassing the deep well, rather than an ‘osculating complex’ that gives rise to the additional forward component. We note that we make a distinction between the direct reaction that avoids the deep potential well, or other cases in which the reaction simply deviates from the minimum energy path [30] , [31] and roaming dynamics that take place following adduct formation. The former dynamics are not unusual in bimolecular reactions: indeed, they were seen in some of the earliest trajectory calculations [32] . Roaming dynamics as shown here and in many unimolecular reactions represent a distinct subset of those reactions that deviate significantly from the minimum energy path. They involve near dissociation, in this case back to reactants, and a TS located at a total potential energy and with vibrational frequencies near those of the reactants or products. This TS then leads to a configuration at which an intramolecular reaction may take place. These are precisely the conditions of the TS seen here, which is analogous to the roaming component in the H+HCO reaction [33] and in many other systems. A comparison of Cl–isobutene to that system, which has been studied using quasiclassical trajectories, is very instructive. For the H+HCO reaction, three outcomes were seen: a direct reaction and complex formation with two decomposition paths: either through a conventional three-centre TS, or by roaming. Both the direct reaction and the roaming reaction give rise to similar high vibrational excitation in the H 2 product. These two pathways are analogous to the direct and indirect reactions seen here, with the exception that in Cl–isobutene there is no three-centre TS for the indirect reaction. In fact, a key difference is that the present system involves a radical and a closed shell molecule exchanging the radical centre along the reaction pathway, giving radical+closed shell products while the H+HCO reaction involves a radical pair giving a pair of closed shell molecules as products. We have recently learned of related work in the Orr-Ewing group at Bristol combining state-resolved velocity map imaging of the HCl product with direct dynamics calculations for this and related systems. Their results clearly support this roaming mechanism as the sole pathway from adduct to products, although they find greater branching for the direct reaction in their experiments than we see here. Preston, T. J. et al. (Personal correspondence). In summary, our experimental results show evidence for the important role played by indirect reactions in the total reaction cross-section of HCl formation in the reaction of Cl with isobutene i -C 4 H 8 . Addition-elimination proceeds through a long-lived complex in which the Cl addition to the double bond is followed by HCl elimination from the adjacent methyl groups. No evidence for a three-centre or four-centre TS is seen in the experimental results, nor in a careful analysis of the ground-state PES. Instead, we find a roaming-type TS located 1–2 kcal mol −1 below the energy of the reactant asymptote with greatly extended C–Cl and Cl–H bond distances and vibrational frequencies very similar to the reactants. The picture is therefore analogous to the roaming mechanism observed previously in unimolecular reactions. In this case the roaming dynamics are central to the addition–elimination reaction mechanism: although abstraction is the only pathway to products, an indirect reaction can occur mediated by the strong electrophilic interaction of the Cl atom with the alkene π cloud. The reactions remain fast and HCl elimination can compete with the Cl loss because of the loose roaming TS combined with the slight enthalpic advantage. Crossed-beam slice imaging experiment The original crossed-beam imaging set-up has been described elsewhere [34] . In the following, we focus on the adopted experimental procedure, along with experimental modifications and improvements relevant for the present study. The two molecular beams were pulsed at 10 Hz with duration of 100 μs by using piezoelectric disk valves and backing pressures of 5 bar. The collision energy was varied by seeding the reactants in H 2 , He, or Ne with <5% dilution. We note the present results for the highest collision energy were found to give improved collision energy definition compared with our earlier study. We used a high-density chlorine radical source that consists in combining Cl 2 photolysis to ablation [35] . For this purpose, the third harmonic of an Nd:YAG laser (355 nm) is focused at the tip of the nozzle, which is embedded in an aluminum extension tube. The same laser pulse generates both photolysis and ablation. The speed ratios, directly measured by imaging the parent beams, are equal to 5 and 8 for Cl 2 /Ne and Cl 2 /He mixtures, respectively. In the reaction chamber, the isobutyl radical products are ionized at 157 nm with an unfocused excimer laser beam. Along the time-of-flight axis, the resulting ion cloud was stretched and accelerated via a four-electrode d.c. slice ion optics assembly to impact on a dual microchannel plate detector coupled to a fast phosphor screen. The front plate of the microchannel plate was held at constant potential, while the back plate ‘gates’ the central slice of the reaction products at a specific m/z ratio by application of a high-voltage pulse. The images were recorded using a CCD camera and the megapixel acquisition programme NuAcq was used to accumulate the raw images containing centroided data [36] . The data presented here are shown after background subtraction and density-to-flux corrections. Background substraction is performed by substracting the velocity-flux maps obtained with the Cl 2 photolysis laser off. These background images show a strong signal at m/z =57, peaking in the forward directions at θ =0° due to the photodissociaton of isobutene by the probe laser that cannot be substracted in the (0–30)° range at E C =14 and 8 kcal mol −1 and in the (0–60)° range at E C =4 kcal mol −1 . Finally, a small density-to-flux correction was performed by scaling the pixel intensity by the lab velocity at each point. Computational methods Ab initio calculations were performed using the CBS-QB3 method [37] implemented in the Gaussian09 quantum chemistry software package [38] , which involves geometry optimization and evaluation of vibrational frequencies at the density functional B3LYP/6-311(2d,d,p) level of theory followed by a series of CCSD(T) and MP2 single-point calculations with various basis sets to extrapolate to the complete basis set limit. Connections between the TS and local minima were verified by IRC calculations at the B3LYP/6-311(2d,d,p) level. The lifetimes of the H 2 CClC(CH 3 ) 2 and H 2 CCCl(CH 3 ) 2 radical complexes were estimated with Rice–Ramsperger–Kassel–Marcus calculations of energy-dependent rate constants for dissociation toward the products in single-collision conditions. The lifetimes of the HCl elimination process from the complexes at collision energies of E C =4, 8 and 14 kcal mol −1 were estimated to be 5, 0.8 and 0.1 ns for H 2 CCCl(CH 3 ) 2 to be compared with 72, 10 and 2 ns for H 2 CClC(CH 3 ) 2 . How to cite this article: Joalland, B. et al. Roaming dynamics in radical addition–elimination reactions. Nat. Commun. 5:4064 doi: 10.1038/ncomms5064 (2014).